Lin28a regulates neuronal differentiation and controls miR-9 production microRNAs shape the identity and function of cells by regulating gene expression. It is known that brain-specific miR-9 is controlled transcriptionally; however, it is unknown whether post-transcriptional processes contribute to establishing its levels. Here we show that miR-9 is regulated transcriptionally and post-transcriptionally during neuronal differentiation of the embryonic carcinoma cell line P19. We demonstrate that miR-9 is more efficiently processed in differentiated than in undifferentiated cells. We reveal that Lin28a affects miR-9 by inducing the degradation of its precursor through a uridylation-independent mechanism. Furthermore, we show that constitutively expressed untagged but not GFP-tagged Lin28a decreases differentiation capacity of P19 cells, which coincides with reduced miR-9 levels. Finally, using an inducible system we demonstrate that Lin28a can also reduce miR-9 levels in differentiated P19 cells. Together, our results shed light on the role of Lin28a in neuronal differentiation and increase our understanding of the mechanisms regulating the level of brain-specific microRNAs. Small (21–22 nucleotide) RNAs called microRNAs (miRs) have emerged as vital regulators of the post-transcriptional control of gene expression [1] . The maturation pathway of miRs, involving nuclear cleavage by the Drosha/DGCR8 complex and cytoplasmic processing by the Dicer complex, has been well described and reviewed [2] , [3] . A mature miR, on entering the miR-induced silencing complex, partially base pairs with target messenger RNA, exerting translational repression and/or mRNA degradation [4] , [5] , [6] . A number of miRs are expressed in a tissue-specific, differentiation or developmental stage-specific manner, thereby contributing to cell identity and function [7] . Importantly, misregulation of miR levels is associated with many pathological conditions, resulting in over or underinhibition of disease-associated genes [8] , [9] , [10] , [11] . Regulation of cellular miR levels is achieved by adjusting their transcription or by modulating post-transcriptional processing events [12] , [13] . However, the contribution of post-transcriptional control to the establishment of the levels of transcriptionally regulated miRs is largely unknown. The human nervous system expresses ~70% of the known miRs, and some of these are specific to neurons [14] . It has been demonstrated that brain-specific miR-9 and miR-124 play an important role in neuronal development [15] , [16] . The expression of miR-9 and miR-124 is transcriptionally regulated by the RE1-silencing transcriptional factor (REST) [17] , [18] . Furthermore, cyclic AMP-response element-binding protein has been shown to promote miR-9 expression [17] . miR-9 is evolutionarily conserved at the nucleotide level but its expression profile and functions are diverse within the nervous system of different species [19] . This miR was shown to interfere with the fibroblast growth factor 8 (ref. 19 ) signalling cascade, an important pathway for neural plate patterning and development of the midbrain–hindbrain boundary [20] . Interestingly, it has been proposed that miR-9 regulates neurogenesis of the mouse telencephalon by orchestrating adjustments in a network of transcription factors [21] . Finally, miR-9 and miR-124 alone can transform adult fibroblasts into neurons, demonstrating their roles as master regulators of neuronal development [22] . We have previously shown that hnRNP A1, a protein implicated in many aspects of RNA processing, binds to the conserved terminal loops (CTLs) of miR-18a (refs 23 , 24 ) and let-7a-1 (ref. 25 ), stimulating and inhibiting processing, respectively. Furthermore, we have identified a number of other primary miR transcripts (including neuro-specific miR-9) with highly CTLs and hypothesized that this may reflect their requirement for auxiliary factors to regulate their processing [24] , [26] , [27] . Recently, we have demonstrated that the brain-enriched expression of miR-7, which is processed from a ubiquitous primary transcript, is supported by inhibition of its biogenesis in non-neural cells [28] . This inhibition is achieved through the HuR-mediated binding of MSI2 to the CTL of the miR-7 primary transcript. The regulation of pri- and pre-let-7 processing by the pluripotency factor Lin28 is an another example of post-transcriptional control of miR levels [29] . It has been well demonstrated that the binding of Lin28a to pre-let-7 induces 3′-terminal uridylation through recruitment of the TUT4 polymerase [30] . This blocks Dicer processing and induces the DIS3L2-mediated degradation of aberrantly processed pre-let-7 transcripts [31] . A number of other miRs have been shown to be under post-transcriptional control [32] . Here we present evidence that the brain-specific miR-9 is regulated not only at the transcriptional level but also post-transcriptionally. We demonstrate that Lin28a, a protein previously implicated in the regulation of let-7 biogenesis, binds to the miR-9 precursor and decreases the cellular levels of miR-9 during retinoic acid (RA)-mediated P19 cell neuronal differentiation. We show that the constitutive expression of untagged but not green fluorescent protein (GFP)-tagged Lin28a causes a severe differentiation phenotype by reducing the size of embryonic bodies. Importantly, the constitutive expression of GFP-tagged Lin28a reduces the levels of let-7a but not miR-9, whereas untagged Lin28 inhibits both miR-9 and let-7a. We reveal that Lin28a controls miR-9 levels by a uridylation-independent mechanism. Finally, using an inducible Tet-On 3G system, we demonstrate that Lin28a can also reduce miR-9 levels in differentiated cells. Our results provide the basis for better understanding the mechanism regulating the levels of brain-specific miRs and their control of neuronal differentiation. Transcriptional and post-transcriptional control of miR-9 To determine whether post-transcriptional regulation of brain-specific miR-9 contributes to establishing its intercellular concentrations, we analysed the level of mature and corresponding primary transcripts at different stages of P19 cell neuronal differentiation. Throughout differentiation, we observed a steady increase in the miR-9 levels to ~50–60-fold on days 4 and 5, reaching ~500–550-fold between days 8 and 10 ( Fig. 1a ). Importantly, the increase in primary miR-9 transcripts was higher at these time points ( Fig. 1b ). On day 4, we observed an ~520-fold increase in pri-miR-9-2, whereas on day 8, pri-miR-9-1, -2 and -3 were induced by ~400-, 1,300- and 260-fold, respectively ( Fig. 1b ). A gradual increase in let-7 and rapid decrease in miR-302a ( Fig. 1c,d ) together with a decrease in Lin28 protein and an increase in the neuronal markers Tuj1 and GFAP ( Supplementary Fig. 1a ) validated an efficient neuronal differentiation phenotype. Northern blot analysis of miR-9, let-7a and miR-302a confirmed their abundance at selected stages of P19 cell neuronal differentiation ( Supplementary Fig. 1b ). Crucially, an unbiased RNAseq and small RNAseq analysis of undifferentiated (day 0) and differentiating (day 4) P19 cells revealed that while primary miR-9-2 levels accumulate from undetectable in d0 to ~900 of normalized reads in d4, the mature miR-9 accumulates very modestly to ~4 normalized reads in d4 ( Supplementary Fig. 2 ). This is in stark contrast with another miR, which is rapidly induced on RA treatment—miR-10a. Primary levels of miR-10a accumulate from undetectable in d0 to ~170 normalized reads in d4. Unlike miR-9, the levels of miR-10a increase from ~4 normalized reads in d0 to ~460 normalized reads in d4 ( Supplementary Fig. 2 ). The levels of control primary and mature miR-16 are much more stable during differentiation. This example clearly demonstrates that miR-9 processing is repressed post-transcriptionally during early stage of neuronal differentiation, whereas miR-10a is most probably free from post-transcriptional regulation. Altogether, these results show that the accumulation of brain-specific miR-9 does not linearly correspond with the changing levels in their primary transcripts. This result suggests the existence of additional post-transcriptional mechanisms regulating the abundance of brain-specific miRs. 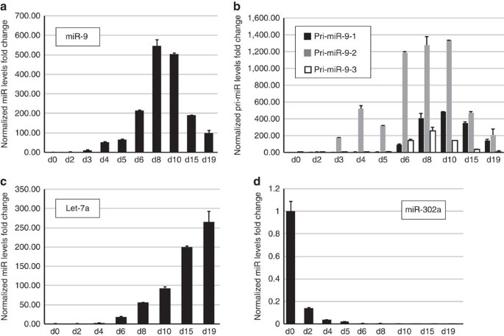Figure 1: The level of brain-specific miR-9 is transcriptionally and post-transcriptionally regulated during RA-induced neuronal differentiation of P19 cells. (a,c,d) Real-time qRT–PCR analysis of mature miR-9, let-7a and miR-302a levels at different stages of RA-induced neuronal differentiation (Day—d). The values were normalized to miR-16 levels. The fold change was plotted relative to values derived from undifferentiated cells (d0), which were set to 1. Mean values and s.d. of three independent biological replicates are shown. (b) Real-time qRT–PCR of miR-9 primary transcripts (pri-miR) at different stages of RA-induced P19 cell neuronal differentiation. The fold changes of the corresponding pri-miRNA abundance, pri-miR-9-1 (black bars), pri-miR-9-2 (grey bars) and pri-miR-9-3 (white bars) were plotted relative to the d0 values, which were set to 1. The values were normalized to the cyclophilin A mRNA levels. Mean values and s.d. of three independent experiments are shown. Figure 1: The level of brain-specific miR-9 is transcriptionally and post-transcriptionally regulated during RA-induced neuronal differentiation of P19 cells. ( a , c , d ) Real-time qRT–PCR analysis of mature miR-9, let-7a and miR-302a levels at different stages of RA-induced neuronal differentiation (Day—d). The values were normalized to miR-16 levels. The fold change was plotted relative to values derived from undifferentiated cells (d0), which were set to 1. Mean values and s.d. of three independent biological replicates are shown. ( b ) Real-time qRT–PCR of miR-9 primary transcripts (pri-miR) at different stages of RA-induced P19 cell neuronal differentiation. The fold changes of the corresponding pri-miRNA abundance, pri-miR-9-1 (black bars), pri-miR-9-2 (grey bars) and pri-miR-9-3 (white bars) were plotted relative to the d0 values, which were set to 1. The values were normalized to the cyclophilin A mRNA levels. Mean values and s.d. of three independent experiments are shown. Full size image miR-9 processing is regulated during neuronal differentiation To determine whether the biogenesis of brain-specific miR-9 is regulated during neuronal differentiation, we employed in vitro processing assays. We observed an accumulation of pre-miR-9-1 and pre-let-7a in pri-miR processing performed in extracts from differentiated cells when compared with those from undifferentiated cells ( Fig. 2 ). Conversely, the processing of pri-miR-302a was more efficient in d0 than in d9 extracts, whereas the in vitro cleavage pattern of pri-miR-101 was more uniform throughout differentiation ( Fig. 2 ). This result suggests that miR-9 processing is regulated by negative or positive factors in undifferentiated and differentiated P19 cells, respectively. Abolished pri-miR-9-1 and pri-let-7a-1 processing in Drosha or DGCR8-depleted HeLa cell extracts confirmed the specificity of the reactions and the molecular weights of the corresponding miR precursors ( Supplementary Fig. 3 ). Interestingly, we observed nonspecific in vitro processing products in d0 extracts for pri-miR-9-1 ( Fig. 2 ) that did not correspond to pre-miRs because they were not detected in processing reactions performed in d9 P19 or HeLa cell extracts ( Fig. 2 and Supplementary Fig. 3 ). Hence, we assumed that the differentiation stage-specific accumulation of pre-miR-9-1 might arise from the regulation of Drosha cleavage or the control of their stability. Together, these observations corroborate our mature miR and pri-miR profiling results, indicating that during neuronal differentiation, the processing of brain-specific miR-9 is regulated at the post-transcriptional level. 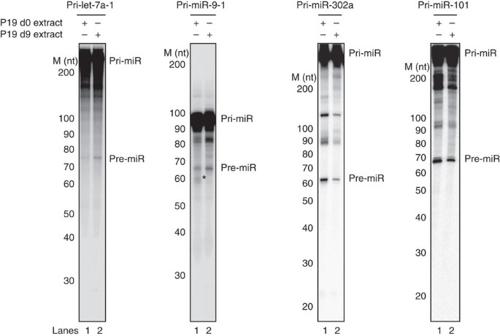Figure 2: Let-7a, miR-9 and miR-302a primary transcripts are differentially processed in undifferentiated and differentiated extracts from P19 cells. Internally radiolabelled primary transcripts (50 × 103c.p.m., ~20 pmol) were incubated in the presence of either d0 (lanes 1) or d9 (lanes 2) P19 cell extracts. The products were analysed on an 8% denaturing polyacrylamide gel. [M], RNA size marker; *, nonspecificin vitroprocessing products. Pri-miR-101 processing served as a control. The results are representative of at least three independent experiments. Figure 2: Let-7a, miR-9 and miR-302a primary transcripts are differentially processed in undifferentiated and differentiated extracts from P19 cells. Internally radiolabelled primary transcripts (50 × 10 3 c.p.m., ~20 pmol) were incubated in the presence of either d0 (lanes 1) or d9 (lanes 2) P19 cell extracts. The products were analysed on an 8% denaturing polyacrylamide gel. [M], RNA size marker; *, nonspecific in vitro processing products. Pri-miR-101 processing served as a control. The results are representative of at least three independent experiments. Full size image Lin28a is a potential regulator of miR-9 biogenesis Conserved terminal loops (CTLs) have been implicated in the regulation of miR biogenesis, and miR-9 has highly conserved terminal loop [24] . Thus, we hypothesized that miR-9 CTL might be involved in the regulation of its processing during neuronal differentiation. To find the putative regulators of miR-9 biogenesis, we used stable isotope labeling with amino acids in cell culture (SILAC) combined with RNA pull down and mass spectrometry ( Fig. 3a ). miR-9 CTL was used to precipitate proteins from extracts derived from undifferentiated (d0) or differentiated (d9) P19 cells that were cultured with heavy [13C]Arg/[13C]Lys or light [12C]Arg/[12Lys] isotopes, respectively. 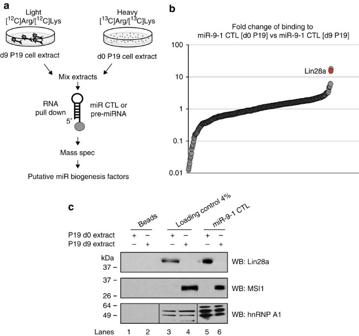Figure 3: SILAC combined with RNA pull down and mass spectrometry reveals putative regulators of brain-specific microRNA biogenesis. (a) Schematic of the method. P19 cells were grown in ‘light’ medium containing12C6-arginine and12C6-lysine or ‘heavy’ medium containing13C6-arginine and13C6-lysine. Cells grown in ‘light’ medium were subjected to RA-induced neuronal differentiation until d9. Next, RNA pull down was performed with agarose beads covalently linked to microRNA CTLs or pre-miRs and incubated with premixed extracts from ‘light’ d9 or ‘heavy’ d0 P19 cells. After RNase treatment, the supernatants were subjected to quantitative mass spectrometry, which identifies putative miR biogenesis factors. (b) The graph represents the fold enrichment of proteins that bind to the miR-9-1 CTL in experiments with ‘heavy’ d0 P19 cell extracts compared with ‘light’ d9 P19 cell extracts. The values are presented on a log10 scale. The Lin28a protein is indicated in red. (c) Western blot analysis of miR-9-1 CTL RNA pull down with d0 and d9 P19 cell extracts for Lin28a, MSI1 and hnRNP A1. Lanes 1 and 2 show reactions with beads alone and d0 and d9 cell extracts, respectively. Lanes 2 and 3 represent 4% (100 μg) of the loading control for d0 and d9 cell extracts, respectively. Lanes 5 and 6 represent miR-9-1 CTL RNA pull downs with d0 and d9 cell extracts, respectively. Lanes 7 and 8 represent miR-9-1 CTL RNA pull downs with d0 and d9 cell extracts, respectively. The results are representative of at least three independent experiments. Figure 3: SILAC combined with RNA pull down and mass spectrometry reveals putative regulators of brain-specific microRNA biogenesis. ( a ) Schematic of the method. P19 cells were grown in ‘light’ medium containing 12 C6-arginine and 12 C6-lysine or ‘heavy’ medium containing 13 C6-arginine and 13 C6-lysine. Cells grown in ‘light’ medium were subjected to RA-induced neuronal differentiation until d9. Next, RNA pull down was performed with agarose beads covalently linked to microRNA CTLs or pre-miRs and incubated with premixed extracts from ‘light’ d9 or ‘heavy’ d0 P19 cells. After RNase treatment, the supernatants were subjected to quantitative mass spectrometry, which identifies putative miR biogenesis factors. ( b ) The graph represents the fold enrichment of proteins that bind to the miR-9-1 CTL in experiments with ‘heavy’ d0 P19 cell extracts compared with ‘light’ d9 P19 cell extracts. The values are presented on a log10 scale. The Lin28a protein is indicated in red. ( c ) Western blot analysis of miR-9-1 CTL RNA pull down with d0 and d9 P19 cell extracts for Lin28a, MSI1 and hnRNP A1. Lanes 1 and 2 show reactions with beads alone and d0 and d9 cell extracts, respectively. Lanes 2 and 3 represent 4% (100 μg) of the loading control for d0 and d9 cell extracts, respectively. Lanes 5 and 6 represent miR-9-1 CTL RNA pull downs with d0 and d9 cell extracts, respectively. Lanes 7 and 8 represent miR-9-1 CTL RNA pull downs with d0 and d9 cell extracts, respectively. The results are representative of at least three independent experiments. Full size image SILAC combined with RNA pull down and mass spectrometry analysis revealed several proteins specifically interacting with miR-9 CTL ( Fig. 3b and Supplementary Data 1 ). Our attention was drawn to the Lin28a protein, a factor implicated in the regulation of let-7 biogenesis, which was highly enriched (17 fold) in pull downs from undifferentiated cells ( Fig. 3b ). We validated the strong interaction between Lin28a and the miR-9-1 CTL ( Fig. 3c ). Crucially, this interaction was observed only in extracts derived from undifferentiated cells. In contrast, the Msi1 protein was found to predominantly interact with the miR-9-1 CTL in differentiated extracts ( Fig. 3c ). The observed interactions were specific because neither Lin28 nor Msi1 interacted with beads alone. Moreover, hnRNP A1, which is a ubiquitous RNA-binding protein, was found to interact equally with corresponding CTLs on days 0 and 9. Indeed, the majority of the identified proteins did not show a differentiation-regulated expression. This, however, does not preclude their potential roles in regulating miR-9 biogenesis. As Lin28a is a potent inhibitor of let-7 biogenesis, we hypothesized that it can also function in the regulation of brain-specific miR biogenesis. To further confirm the interactions, we performed SILAC combined with pre-miR pull down and mass spectrometry using extracts from undifferentiated P19 cells. Pre-let-7a pull down identified Lin28a as well as Khsrp and hnRNP A1, proteins previously implicated in the regulation of let-7 biogenesis [25] , [33] , [34] ( Supplementary Table 1 and Supplementary Data 2 ). Surprisingly, we did not find TuT4 in the pre-let-7a pull down, suggesting that the Lin28a/TuT4 interaction might be transient under our experimental conditions ( Supplementary Data 2 ). Full-length pre-miR-9-1 and pre-miR-9-2 pulled down Lin28 with fold enrichment similar to that observed for pre-let-7a. The pre-miR-9 pull down revealed a number of other specific factors that may contribute to the regulation of miR-9 processing. To validate Lin28a-binding specificity, we performed RNA pull down followed by western blot analysis with a panel of pre-miRs. Pre-miR-9-1, pre-let-7a-1 and pre-miR-101 displayed efficient Lin28a binding ( Fig. 4a ). Importantly, pre-miR-16 as well as pre-miR-9-1 with substituted TL from the miR-16 (pre-miR-9-1/miR-16 TL) could not pull down Lin28a ( Fig. 4a ). This was also confirmed by electrophoretic mobility shift assay (EMSA) analysis of pre-miRs and anti-Lin28a antibody ( Fig. 4b ). In EMSA, pre-miR-9-1 as well as pre-let-7a-1 form several complexes with proteins from d0 P19 cell extracts. Formation of one of the complexes is abolished on addition of anti-Lin28a but not unspecific antibody ( Fig. 4b ). This suggests that Lin28a bound to pre-miR-9-1 and pre-let-7a-1 forms a complex with the anti-Lin28a antibody, preventing the substrates to enter the gel. Alternatively, anti-Lin28a antibody could be binding to Lin28a and precluding its association with its substrates. Importantly, pre-miR-16 was not shifted in undifferentiated cell extracts. This provides additional evidence for the specificity of Lin28a binding. 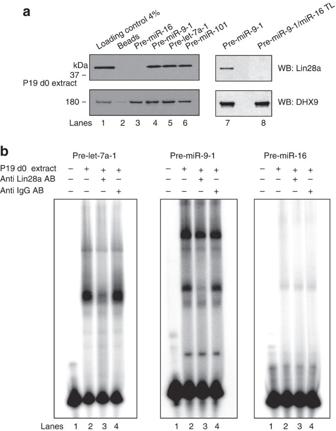Figure 4: Lin28a binds specifically to pre-miRs. (a) Western blot analysis of pre-miR pull down with d0 P19 cell extracts for Lin28a and DHX9. Lane 1 represents 4% (100 μg) of the loading control. Lane 2 shows reactions with beads alone, lane 3 with pre-miR-16, lanes 4 and 7 with pre-miR-9-1, lane 5 with pre-let-7a-1, lane 6 with pre-miR-101 and lane 8 with pre-miR-9-1/miR-16 TL mutant. (b) EMSA analysis of pre-miRs in extracts from d0 P19 cells. Where indicated, 1:100 of antibody was added to reaction mixture. Lane 1 represents controls without added extract, lane 2 with d0 extracts, lane 3 with d0 extract and anti-Lin28a antibody and lane 4 with d0 and anti IgG antibody. The results are representative of at least three independent experiments. Figure 4: Lin28a binds specifically to pre-miRs. ( a ) Western blot analysis of pre-miR pull down with d0 P19 cell extracts for Lin28a and DHX9. Lane 1 represents 4% (100 μg) of the loading control. Lane 2 shows reactions with beads alone, lane 3 with pre-miR-16, lanes 4 and 7 with pre-miR-9-1, lane 5 with pre-let-7a-1, lane 6 with pre-miR-101 and lane 8 with pre-miR-9-1/miR-16 TL mutant. ( b ) EMSA analysis of pre-miRs in extracts from d0 P19 cells. Where indicated, 1:100 of antibody was added to reaction mixture. Lane 1 represents controls without added extract, lane 2 with d0 extracts, lane 3 with d0 extract and anti-Lin28a antibody and lane 4 with d0 and anti IgG antibody. The results are representative of at least three independent experiments. Full size image The knockdown of Lin28a leads to increased levels of miR-9 Lin28a expression is dynamically regulated throughout neuronal differentiation [33] . Its expression is elevated at early stages of development and is switched off during differentiation. This regulation is essential for the inhibition of let-7 production at the early stages of differentiation and development and for maintaining pluripotency [33] , [35] . We observed a steady decrease in Lin28 until day 6 and a sharp drop in its expression on day 8 ( Supplementary Fig. 1a ). This decline coincided with a sharp increase in miR-9 levels on day 8, although a substantial accumulation of primary miR-9 transcripts occurs at earlier stages of neuronal differentiation ( Fig. 1a,b ). To determine whether Lin28a controls miR-9 levels, we transfected P19 cells with anti-Lin28a short interfering RNAs (siRNAs). To initiate miR-9 expression, we then induced transfected cells to differentiate. Western blot analysis of Lin28a expression on day 4 of differentiation demonstrated that the protein was depleted to ~20–30% of control treatment ( Fig. 5a ). As expected, Lin28a depletion resulted in a fourfold increase in let-7a levels ( Fig. 5b ). The level of miR-101 and miR-122, miRs unrelated to neuronal development, was unchanged. Crucially, Lin28a knockdown resulted in a modest but statistically significant 1.6-fold increase in miR-9 levels on day 4 of P19 neuronal differentiation ( Fig. 5b ). 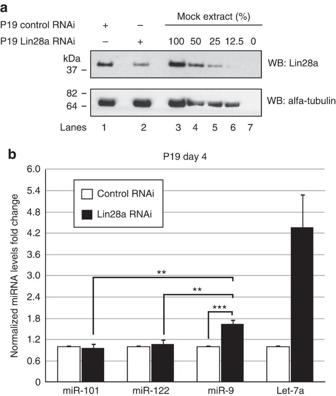Figure 5: Lin28a regulates miR-9 levels differentiating P19 cells. (a) Western blot analysis of protein extracts from mock-depleted P19 cells (lane 1) and Lin28a-depleted P19 cells (lane 2). Lanes 3 through 7 show serial dilutions of total protein extracts from mock-depleted P19 cells, providing an estimation of the linearity of the western blot assay and the limit of detection. (b) Real-time qRT–PCR analysis of the mature miR-101, miR-122, miR-9 and let-7a levels on day 4 (d4) of RA-induced neuronal differentiation. The results from the mock-depleted cells are shown as white bars; the results from Lin28a-depleted cells are shown as black bars. The values were normalized to the miR-16 level. The fold change was plotted relative to values derived from mock-depleted cells, which were set to 1. Mean values and s.d. of three independent biological replicates are shown. Statistical significance was calculated usingt-test; **P⩽0.01; ***P⩽0.001. Figure 5: Lin28a regulates miR-9 levels differentiating P19 cells. ( a ) Western blot analysis of protein extracts from mock-depleted P19 cells (lane 1) and Lin28a-depleted P19 cells (lane 2). Lanes 3 through 7 show serial dilutions of total protein extracts from mock-depleted P19 cells, providing an estimation of the linearity of the western blot assay and the limit of detection. ( b ) Real-time qRT–PCR analysis of the mature miR-101, miR-122, miR-9 and let-7a levels on day 4 (d4) of RA-induced neuronal differentiation. The results from the mock-depleted cells are shown as white bars; the results from Lin28a-depleted cells are shown as black bars. The values were normalized to the miR-16 level. The fold change was plotted relative to values derived from mock-depleted cells, which were set to 1. Mean values and s.d. of three independent biological replicates are shown. Statistical significance was calculated using t -test; ** P ⩽ 0.01; *** P ⩽ 0.001. Full size image To uncouple the effects of differentiation and control of miR-9 levels, we performed pri-miR transgene overexpression in undifferentiated P19 cells. Overexpression of pri-miR-9 and pri-let-7a driven by a cytomegalovirus (CMV) promoter resulted in a very small induction of mature miRs ( Supplementary Fig. 4 ). Importantly, overexpression of pri-let-7a-1/miR-16 TL mutant, which escapes Lin28a-mediated regulation, produced more than 20-fold mature let-7a. This suggests that the accumulation of miR-9 and let-7a levels in undifferentiated cells is post-transcriptionally suppressed. Interestingly, overexpression of cognate pri-miR-9-1/miR-16 TL mutant did not result in de-repression of miR-9 accumulation ( Supplementary Fig. 4 ). This implies the existence of additional layers of post-transcriptional miR-9 regulation, most probably preventing accumulation of mature miR in undifferentiated cells. All these results suggest that Lin28a expression has an influence on the level of miR-9 in vivo . The difference between the observed effects of Lin28 depletion on the miR-9 and let-7 levels could be due to different levels of corresponding primary transcripts available at early stages of differentiation. The expression of the let-7 primary transcript is stable throughout differentiation, whereas the miR-9 primary transcript is not detected in undifferentiated P19 cells and only begins to accumulate during early stages of neuronal differentiation [17] . Together, these results provide evidence implicating Lin28a in the regulation of brain-specific miR-9 abundance during neuronal differentiation. Untagged Lin28a affects miR-9 and neuronal differentiation Next, we wanted to determine whether prolonged expression of Lin28a during neuronal differentiation could affect the level of let-7a and miR-9. To test this hypothesis, P19 cells constitutively expressing untagged or GFP-tagged Lin28a together with the relevant control cell lines were subjected to RA-induced neuronal differentiation. Western blot analysis of untagged and GFP-tagged Lin28a confirmed their prolonged expression throughout P19 differentiation ( Fig. 6a,b ). During the differentiation of P19 cells constitutively expressing untagged Lin28a, we observed a significant reduction in the size of embryonic bodies ( Fig. 6c,d ). Surprisingly, P19 cells with stable Lin28a-GFP expression were phenotypically indistinguishable from control P19 cell lines. This result indicates that GFP-tagged Lin28a does not confer all of the functions of the wild-type protein. Indeed, prolonged GFP-Lin28a expression during neuronal differentiation resulted in an approximately fourfold decrease in let-7a compared with control cells but had no significant effect on the level of miR-9 ( Fig. 6e ). 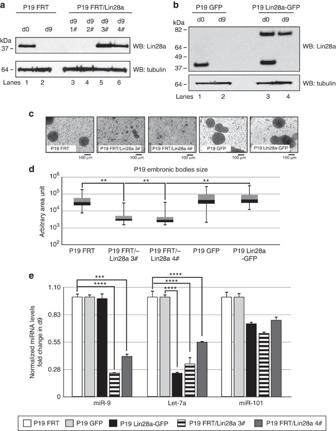Figure 6: Constitutive expression of untagged but not GFP-tagged Lin28a affects miR-9 biogenesis during P19 cell differentiation. (a) Western blot analysis of Lin28a levels in P19 stable cell lines expressing untagged human Lin28a. Lanes 1 and 2 include d0 and d9 P19 cells with an integrated FRT site, respectively. Lanes 3 and 4 show the P19 FRT/Lin28a clone, which does not express Lin28a at day 9. Lanes 5 and 6 include P19 FRT/Lin28a clones with stable Lin28a expression in differentiated cells. Tubulin served as a loading control. (b) Western blot analysis of the Lin28a levels in P19 stable cell lines expressing GFP-tagged human Lin28a. Lanes 1 and 2 are d0 and d9 P19 cells with integrated GFP, respectively. Lanes 3 and 4 are P19 Lin28a-GFP cell lines with stable expression of GFP-tagged human Lin28a in undifferentiated and differentiated cells, respectively. Tubulin served as a loading control. (c) Bright-field microscopy images showing representative images of P19 embryonic bodies at day 4 of differentiation. (d) Quantification of P19 embryonic bodies sizes at day 4 of differentiation represented as box plots. Statistical significance was calculated using the Mann–WhitneyU-test; **P⩽0.01; ***P⩽0.001. (e) Real-time qRT–PCR analysis of mature miR-9, let-7a and miR-101 on day 9 of P19 FRT (white bars), P19 GFP (light grey bars), P19 GFP-Lin28a (black bars), P19 FRT/Lin28a 3# (horizontal lines bars) and P19 FRT/Lin28a 4# (dark grey bars). The values were normalized to miR-16 levels. The fold change was plotted relative to values derived from the corresponding control cell lines P19 FRT and P19 GFP, which were set to 1. Mean values and s.d. of three independent biological replicates are shown. Statistical significance was calculated usingt-test; ***P⩽0.001; ****P⩽0.0001. Figure 6: Constitutive expression of untagged but not GFP-tagged Lin28a affects miR-9 biogenesis during P19 cell differentiation. ( a ) Western blot analysis of Lin28a levels in P19 stable cell lines expressing untagged human Lin28a. Lanes 1 and 2 include d0 and d9 P19 cells with an integrated FRT site, respectively. Lanes 3 and 4 show the P19 FRT/Lin28a clone, which does not express Lin28a at day 9. Lanes 5 and 6 include P19 FRT/Lin28a clones with stable Lin28a expression in differentiated cells. Tubulin served as a loading control. ( b ) Western blot analysis of the Lin28a levels in P19 stable cell lines expressing GFP-tagged human Lin28a. Lanes 1 and 2 are d0 and d9 P19 cells with integrated GFP, respectively. Lanes 3 and 4 are P19 Lin28a-GFP cell lines with stable expression of GFP-tagged human Lin28a in undifferentiated and differentiated cells, respectively. Tubulin served as a loading control. ( c ) Bright-field microscopy images showing representative images of P19 embryonic bodies at day 4 of differentiation. ( d ) Quantification of P19 embryonic bodies sizes at day 4 of differentiation represented as box plots. Statistical significance was calculated using the Mann–Whitney U -test; ** P ⩽ 0.01; *** P ⩽ 0.001. ( e ) Real-time qRT–PCR analysis of mature miR-9, let-7a and miR-101 on day 9 of P19 FRT (white bars), P19 GFP (light grey bars), P19 GFP-Lin28a (black bars), P19 FRT/Lin28a 3# (horizontal lines bars) and P19 FRT/Lin28a 4# (dark grey bars). The values were normalized to miR-16 levels. The fold change was plotted relative to values derived from the corresponding control cell lines P19 FRT and P19 GFP, which were set to 1. Mean values and s.d. of three independent biological replicates are shown. Statistical significance was calculated using t -test; *** P ⩽ 0.001; **** P ⩽ 0.0001. Full size image Strikingly, constitutive expression of untagged Lin28a resulted in a significant reduction in the miR-9 and let-7a levels at the final stages of P19 cell neuronal differentiation ( Fig. 6e ). Similar results were obtained from two independent Lin28a integrations. The western blot of Lin28a on extracts from differentiated P19 FRT/Lin28a and P19 Lin28a/GFP cells revealed similar levels of GFP-tagged and untagged Lin28a ( Supplementary Fig. 5 ). Thus, the observed phenotypic and functional differences arose from qualitative but not quantitative differences between tagged and untagged Lin28a. The level of primary miR-9 transcripts was also decreased in P19 cells constitutively expressing untagged Lin28a, corroborating the existence of a negative feedback loop between miR-9 and the REST complex, which controls miR-9 expression and is reciprocally controlled by miR-9 ( Supplementary Fig. 6 ). Together, these are important observations for two reasons: they validate Lin28a as a regulator of miR-9 levels and they suggest that GFP-tagged Lin28a could be functionally compromised. Finally, our results provide evidence that the mechanism of Lin28a-mediated miR biogenesis inhibition might be different for let-7 and miR-9. Pre-miR-9 is destabilized in early stages of differentiation It is well documented that Lin28a inhibits members of the let-7 family at the early stages of differentiation and development through recruitment of TuT4 (or TuT7), which uridylates pre-let-7 and leads to its degradation by DIS3L2-mediated pre-let-7 degradation [30] , [31] , [36] . Our in vivo data suggest that Lin28a could inhibit miR-9 through a different mechanism because untagged Lin28a impairs miR-9 and let-7 processing, whereas only let-7 is affected by expression of the GFP-tagged Lin28a. To determine whether pre-miR-9 is regulated in a manner different from pre-let-7, we performed in vitro uridylation assays in P19 cell extracts from subsequent stages of neuronal differentiation. Pre-let-7a was efficiently uridylated in extracts derived from undifferentiated P19 cells ( Fig. 7a ). The intensity of the band corresponding to the uridylated form of pre-let-7a was reduced in reactions with extracts isolated from subsequent stages of neuronal differentiation ( Fig. 7a ). This reduction resulted in a small but significant increase in the stability of the pre-let-7a probe ( Fig. 7c ). In contrast, pre-miR-9 was not converted to a uridylated form but instead was significantly destabilized in extracts derived from undifferentiated P19 cells ( Fig. 7a,c ). 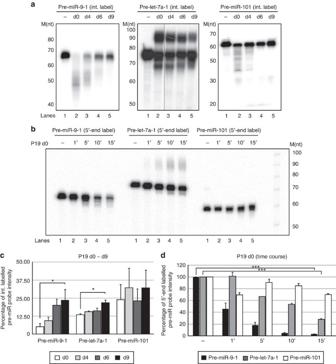Figure 7: Pre-miR-9 is destabilized in P19 cell extracts from the early stages of neuronal differentiation. (a)In vitroprocessing assays were performed with internally radiolabelled pre-miR transcripts (50 × 103c.p.m., ~20 pmol) in the presence of d0 (lanes 2), d4 (lanes 3), d6 (lanes 4) or d9 (lanes 4) P19 cell extracts. (−) represents an untreated control. Reactions were supplemented with 0.25 mM UTP. The products were analysed on an 8% denaturing polyacrylamide gel. [M], RNA size marker. (b)In vitroprocessing assays were performed with 5′-end-labelled pre-miR transcripts (50 × 103c.p.m., ~20 pmol). Pre-miRs were incubated in d0 P19 cell extracts for 1 (1′), 5 (5′), 10 (10′) or 15 min (15′). The control (−) was incubated without extract for 15′. [M], RNA size marker. (c,d) The percentage of pre-miR substrate intensity remaining after correspondingin vitroprocessing reactions was plotted relative to the control reactions set to 100. Mean values and s.d. of three independent experiments are shown. Statistical significance was calculated using at-test; *P⩽0.05; ***P⩽0.001. Figure 7: Pre-miR-9 is destabilized in P19 cell extracts from the early stages of neuronal differentiation. ( a ) In vitro processing assays were performed with internally radiolabelled pre-miR transcripts (50 × 10 3 c.p.m., ~20 pmol) in the presence of d0 (lanes 2), d4 (lanes 3), d6 (lanes 4) or d9 (lanes 4) P19 cell extracts. (−) represents an untreated control. Reactions were supplemented with 0.25 mM UTP. The products were analysed on an 8% denaturing polyacrylamide gel. [M], RNA size marker. ( b ) In vitro processing assays were performed with 5′-end-labelled pre-miR transcripts (50 × 10 3 c.p.m., ~20 pmol). Pre-miRs were incubated in d0 P19 cell extracts for 1 (1′), 5 (5′), 10 (10′) or 15 min (15′). The control (−) was incubated without extract for 15′. [M], RNA size marker. ( c , d ) The percentage of pre-miR substrate intensity remaining after corresponding in vitro processing reactions was plotted relative to the control reactions set to 100. Mean values and s.d. of three independent experiments are shown. Statistical significance was calculated using a t -test; * P ⩽ 0.05; *** P ⩽ 0.001. Full size image Significantly, incubation of pre-miR-9 with extracts derived from days 4, 6 and 9 resulted in its gradual stabilization by two-, four- and fivefold, respectively, which correlates with the period when Lin28a expression is reduced. Pre-miR-9-2 and pre-miR-9-3 are also destabilized in extract derived from d0 P19 cells ( Supplementary Fig. 7 ). Importantly, pri-miR-9-1/miR-16 TL mutant, which does not bind Lin28a ( Fig. 4a ), is not destabilized in extracts from undifferentiated cells ( Supplementary Fig. 7 ). Control pre-miR-101 and pre-let-7a probes were more stable under similar conditions ( Fig. 7a,c ). To establish how pre-miR-9 is degraded, we incubated 5′-end-labelled miR precursors in d0 extracts. Pre-miR-9-1 is more unstable than pre-let-7a and pre-miR-101, showing signs of 3′–5′ and 5′–3′ degradation ( Fig. 7b,d ). These results validate our in vivo data and point to different mechanisms by which miR-9 and let-7a levels are post-transcriptionally regulated during neuronal differentiation. Lin28a destabilizes pre-miR-9 independently of uridylation Thus far, we have shown that Lin28a can bind to the miR-9 CTL and influence miR-9 cellular levels. In addition, we have demonstrated that pre-miR-9 is rendered unstable in P19 cell extracts by a mechanism that is different than that for pre-let-7. To determine whether Lin28a mediates the observed destabilization of pre-miR-9 in undifferentiated cells, we performed pre-miR-processing assays in P19 cell extracts with depleted Lin28a. Incubation of pre-let-7a with Lin28a-depleted extracts resulted in a reduction in pre-let-7a uridylation ( Fig. 8a ). The pre-miR-9 substrate was significantly stabilized in Lin28a-depleted extracts when compared with control ( Fig. 8a,b ). In similar conditions, the level of pre-miR-101 remained largely unchanged ( Fig. 8a,b ). Similarly, degradation of 5′-end-labelled pre-miR-9-1 was strongly suppressed in Lin28a RNAi-depleted P19 d0 extracts compared with reactions in control RNAi extracts ( Supplementary Fig. 8 ). 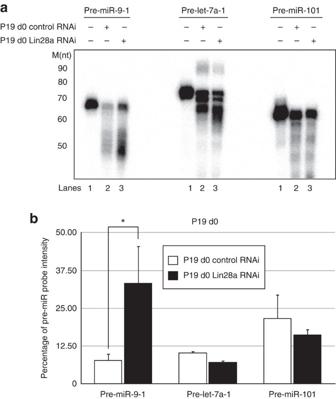Figure 8: Pre-miR-9 is stabilized in Lin28a-depleted P19 cell extracts. (a)In vitroprocessing assays were performed with internally radiolabelled pre-miR transcripts (50 × 103c.p.m., ~20 pmol) in the presence of either mock-depleted (lanes 2, 5, 8) or Lin28a-depleted (lanes 3, 6, 9) d0 P19 cell extracts. (−) represents the untreated control (lanes 1, 4, 7). Reactions were supplemented with 0.25 mM UTP. The products were analysed on an 8% denaturing polyacrylamide gel. (b) The percentage of pre-miR substrate intensity remaining after correspondingin vitroprocessing reactions was plotted relative to the control reactions set to 100. Mean values and s.d. of three experimental replicates are shown. Statistical significance was calculated using at-test; *P⩽0.05. Figure 8: Pre-miR-9 is stabilized in Lin28a-depleted P19 cell extracts. ( a ) In vitro processing assays were performed with internally radiolabelled pre-miR transcripts (50 × 10 3 c.p.m., ~20 pmol) in the presence of either mock-depleted (lanes 2, 5, 8) or Lin28a-depleted (lanes 3, 6, 9) d0 P19 cell extracts. (−) represents the untreated control (lanes 1, 4, 7). Reactions were supplemented with 0.25 mM UTP. The products were analysed on an 8% denaturing polyacrylamide gel. ( b ) The percentage of pre-miR substrate intensity remaining after corresponding in vitro processing reactions was plotted relative to the control reactions set to 100. Mean values and s.d. of three experimental replicates are shown. Statistical significance was calculated using a t -test; * P ⩽ 0.05. Full size image To further demonstrate the role of Lin28a in controlling pre-miR-9 stability, we performed in vitro processing in extracts derived from cell lines with constitutive Lin28a expression. Similar to wild-type, d9 extracts derived from P19 cells stably expressing Lin28a-GFP support degradation of pre-miR-9-1 ( Supplementary Fig. 9a,b ). Pre-let-7a is uridylated in extracts from d0 and d9 derived from both P19 Lin28a-GFP and P19/FRT Lin28a cells. Notably, pre-miR-9-1 is not stabilized in d9 extracts derived from cells constitutively expressing untagged Lin28a ( Supplementary Fig. 9a,b ). These results further support the role of Lin28a in pre-miR-9 destabilization, which leads to decreased cellular levels of miR-9. Since in vitro processing reactions are uncoupled from the effects of transcription, the above results suggest that Lin28a can regulate pre-miR-9 post-transcriptionally. Induced Lin28a in differentiated cells downregulates miR-9 To test whether in vivo regulation of miR-9 by Lin28a is achievable after the cells have been differentiated, we created Tet-On 3G P19 cells that express Lin28a under a doxycycline (Dox)-inducible CMV promoter. Selected clones were subjected to RA-mediated differentiation and programmed with Dox at day 8 of differentiation, when the miR-9 levels approach maximum ( Fig. 1 ). The cells were harvested at day 9 and compared with uninduced cells from the corresponding clones. One of the analysed clones (P19 Tet-On 3G Lin28a 3#) showed induction of Lin28a on Dox treatment ( Fig. 9 ); albeit the levels were much lower when compared with undifferentiated cells. Crucially, only this clone, but not those that did not induce Lin28a, showed a specific downregulation of miR-9 and let-7a levels ( Fig. 9b ). The levels of pri-miR-9 transcripts were also decreased on Dox treatment ( Fig. 9b ), suggesting that Lin28a can directly or indirectly influence the abundance of primary miR-9. Notably, pri-let-7a-1 levels were upregulated supporting the previously suggested role of Lin28a in repressing pri-let-7a-1 Drosha cleavage. 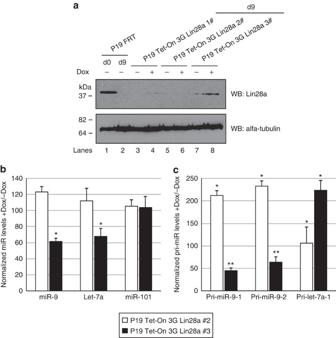Figure 9: Lin28a induction in differentiated P19 cells results in reduction of miR-9 levels. (a) Western blot analysis of protein extracts from control P19 cells (lane 1—d0 and lane 2—d9) and d9 of three colonies of P19 Tet-On 3G Lin28a cells. Lanes 3, 5 and 7 represent results from the corresponding cell lines without Dox. Lanes 4, 6 and 8 show results from the corresponding cell lines induced with Dox (100 ng ml−1). (b) Real-time qRT–PCR analysis of mature miR-9, let-7a and miR-101 levels of Dox-induced cells after RA-mediated neuronal differentiation. The results from P19 Tet-On 3G Lin28a #2, which failed to induce Lin28a, is shown as white bars; the results from P19 Tet-On 3G Lin28a #3, which induced Lin28a, are shown as black bars. The values were normalized to miR-16 levels. The fold change was plotted relative to values derived from −Dox cells, which were set to 100. Mean values and s.d. of three independent biological replicates are shown. Statistical significance was calculated usingt-test; *P⩽0.05. (c) Real-time qRT–PCR analysis of the primary miR-9-1, miR-9-2 and let-7a-1 of Dox-induced cells after RA-mediated neuronal differentiation. The results from P19 Tet-On 3G Lin28a #2, which failed to induce Lin28a, is shown as white bars; the results from P19 Tet-On 3G Lin28a #3, which induced Lin28a, are shown as black bars. The values were normalized to cyclophilin A mRNA levels. Mean values and s.d. of three independent experiments are shown; *P⩽0.05; **P⩽0.01. Figure 9: Lin28a induction in differentiated P19 cells results in reduction of miR-9 levels. ( a ) Western blot analysis of protein extracts from control P19 cells (lane 1—d0 and lane 2—d9) and d9 of three colonies of P19 Tet-On 3G Lin28a cells. Lanes 3, 5 and 7 represent results from the corresponding cell lines without Dox. Lanes 4, 6 and 8 show results from the corresponding cell lines induced with Dox (100 ng ml −1 ). ( b ) Real-time qRT–PCR analysis of mature miR-9, let-7a and miR-101 levels of Dox-induced cells after RA-mediated neuronal differentiation. The results from P19 Tet-On 3G Lin28a #2, which failed to induce Lin28a, is shown as white bars; the results from P19 Tet-On 3G Lin28a #3, which induced Lin28a, are shown as black bars. The values were normalized to miR-16 levels. The fold change was plotted relative to values derived from −Dox cells, which were set to 100. Mean values and s.d. of three independent biological replicates are shown. Statistical significance was calculated using t -test; * P ⩽ 0.05. ( c ) Real-time qRT–PCR analysis of the primary miR-9-1, miR-9-2 and let-7a-1 of Dox-induced cells after RA-mediated neuronal differentiation. The results from P19 Tet-On 3G Lin28a #2, which failed to induce Lin28a, is shown as white bars; the results from P19 Tet-On 3G Lin28a #3, which induced Lin28a, are shown as black bars. The values were normalized to cyclophilin A mRNA levels. Mean values and s.d. of three independent experiments are shown; * P ⩽ 0.05; ** P ⩽ 0.01. Full size image All our results support specific binding of Lin28a to the miR-9 CTL and its role in regulating cellular miR-9 levels. Our data strongly suggest that pre-miR-9 is regulated transcriptionally and post-transcriptionally by a Lin28a-mediated degradation mechanism. These results pave the way to further in-depth analysis required to determine the fine details of Lin28a-mediated control of miR-9, and towards better understanding of Lin28a contribution to neuronal function and differentiation. The biogenesis of miRs is a multistep process that needs to be finely regulated, reflecting their many important roles in animal cells. Despite extensive research in the biological functions of miRs, little is known about the post-transcriptional mechanisms controlling their abundance. In many cases, the levels of primary miR transcripts are not correlated with the absolute levels of corresponding mature miRs [37] . In these cases, post-transcriptional regulation of miR processing is predicted to play a major role in controlling the level of the miRs in question [2] , [38] , [39] . For example, during neuronal differentiation, the let-7 levels are negatively correlated with the expression of Lin28 but display no correlation with its corresponding primary transcripts [40] . Similar observations have been made during the development of Caenorhabditis elegans [41] . In addition, the biogenesis of brain-enriched miR-7, which is produced from a ubiquitous primary transcript, is inhibited by the HuR/MSI2 complex in non-neuronal cells [28] . Our current study shows that the levels of neuro-specific miR-9, which is responsible for neuronal development, undergo extensive transcriptional and post-transcriptional regulation. miR-9 is transcriptionally suppressed by the anti-neural REST complex [17] , [18] . During neuronal differentiation, miR-9 target components of REST, allowing their own expression and that of other neuronal genes. In addition, miR-9 promotes neural cell differentiation by targeting the TLX nuclear receptor, which is responsible for the maintenance of self renewal [42] . In accordance with previous findings, we observed an increase in the level of miR-9 during RA-induced neuronal differentiation in P19 cells [43] . At the early stages of differentiation, the accumulation of the three miR-9 primary transcripts substantially exceeded the accumulation of mature miR-9. These results point to the existence of previously uncharacterized post-transcriptional mechanisms regulating the intercellular levels of miR-9. Using SILAC coupled with RNA pull down and mass spectrometry [28] , we identified several putative regulators of miR-9. We isolated Lin28a as a factor binding to the miR-9 CTL in undifferentiated P19 cells. It is believed that let-7 family members are the main miRs regulated by Lin28 during neuronal differentiation [44] . During muscle differentiation, Lin28 and MBNL1 control miR-1 biogenesis through a uridylation-dependent mechanism [45] . An AGGAG consensus sequence was previously found to be crucial for the association between the Zn-knuckle domain of Lin28a and the let-7 CTL [46] . The miR-9 CTL has a GGAG motif, which can provide a platform for interaction with Lin28a. However, other U-rich sequences were shown to interact with Lin28a through its cold shock domain [29] . In accordance with these observations, pre-miR-9-1 and pre-miR-9-2 were shown to bind recombinant Lin28a in vitro [47] . Interestingly, several studies have used crosslinking and immunoprecipitation coupled with high-throughput sequencing (CLIP-seq) to identify targets for Lin28a binding but failed to detect miR-9 precursors [48] , [49] . These studies focused on undifferentiated embryonic stem cells and somatic cells. Therefore, it is plausible that such an approach could result in a failure to capture targets that are dynamically regulated throughout differentiation. The constitutive expression of untagged Lin28a during neuronal differentiation resulted in a severe differentiation phenotype characterized by small embryonic bodies and reduced levels of mature miR-9 and let-7a. Previously, it has been reported that constitutive expression of Lin28-GFP inhibits let-7a processing in P19 cells and results in a neuronal phenotype that is independent of let-7 (ref. 35 ). Unexpectedly, constitutive expression of a Lin28a-GFP-tagged protein resulted in efficient reduction of let-7a but not miR-9 levels. Similarly, a severe differentiation phenotype was only evident in P19 cells constitutively expressing untagged but not GFP-tagged Lin28a protein. Notably, it has been shown that miR-9 depletion also results in a severe differentiation phenotype characterized by small embryonic bodies, which corroborates our results [50] . First, these findings suggest that decreased let-7 levels are not sufficient to induce an aberrant P19 differentiation phenotype. Second, the mechanisms for Lin28a-mediated inhibition of miR-9 and let-7 are different. Our in vitro processing results, obtained from the wild-type cells and cells constitutively expressing Lin28a, indicate that Lin28a destabilizes pre-miR-9 but does not induce uridylation as observed for pre-let-7 transcripts [30] . Furthermore, induction of Lin28a expression in differentiated cells leads to reduction of miR-9 levels, arguing that the Lin28a control over miR-9 is not restricted to differentiating cells. Further in-depth analysis is required to determine the effectors of the Lin28a-mediated control of pre-miR-9 stability and understand their contribution to neuronal differentiation. miR-9 and miR-124 have been shown to be master regulators of neuronal programs because they alone can transform adult fibroblasts into neurons [22] . We hypothesize that their highly restricted, brain-specific expression profile needs to be safeguarded by several non-mutually exclusive mechanisms. Here we show that miR-9 is transcriptionally and post-transcriptionally controlled. We present evidence that untagged Lin28a inhibits miR-9 processing by destabilizing pre-miR-9 through a uridylation-independent mechanism. This finding sheds more light on the role of Lin28a in neuronal differentiation. Altogether, our results demonstrate that transcriptionally regulated miRs can undergo complementary post-transcriptional control. This has important implications for the understanding of how miRs are regulated and the development of novel miR-based compounds and therapeutics. Cell culture and neuronal differentiation conditions Mouse teratocarcinoma P19 cells or HeLa cells (the American Type Culture Collection) were maintained in standard DMEM medium (Life Technologies), supplemented with 10% fetal bovine serum (Life Technologies). All-trans RA (Sigma) was used to induce neuronal differentiation. In brief, ~12 × 10 6 cells were plated on a non-adhesive dish in DMEM supplemented with 5% serum and supplemented with 1 μM of RA. This induced the formation of embryonic bodies. After 4 days, the embryonic bodies were re-suspended in DMEM supplemented with 10% serum and re-plated on an adhesive dish. Differentiation was followed up to 19 days post induction. At d9, cells displayed neuronal-like morphology. For SILAC mass spectrometry, undifferentiated cells were cultured in DMEM supplemented with ‘heavy’ [ 13 C]Arg/[ 13 C]Lys isotopes and differentiation was performed using DMEM supplemented with ‘light’ [ 12 C]Arg/[ 12 Lys] isotopes (Pierce SILAC Proteins Quantitation Kit, Thermo Scientific). Real-time qRT–PCR and miRNA qRT–PCR analysis Real-time quantitative reverse transcription (qRT)–PCR was performed using the SuperScript III Platinum SYBR Green One-Step qRT–PCR Kit (Life Technologies) following the manufacturer’s instructions on a Roche 480 LightCycler. Generally, 1 μl (500 ng) of total RNA isolated with TRIzol (Life Technologies) was used in a 20-μl reaction, and each sample was run in duplicate. To assess the levels of the corresponding transcripts, values were normalized to cyclophilin A mRNA levels. For each measurement, three independent experiments were performed. Primers are listed in Supplementary Table 4 . miR qRT–PCR analysis was performed using the miSript qRT–PCR kit (Qiagen) on total RNA isolated with TRIzol (Life Technologies) and each sample was run in duplicate. To assess the levels of the corresponding miRs, values were normalized to miR-16. For each measurement, three independent experiments were performed. Northern blot analysis Twenty micrograms of total RNA was mixed with an equal volume of loading buffer (95% formamide, 18 mM EDTA, 0.025% SDS, xylene cyanol, bromophenol blue) and resolved on a 10% PAGE–Urea gel. The ribosomal RNA was visualized with ethidium bromide to confirm equal loading. The RNA was transferred from the gel onto nitrocellulose membrane (Hybond N). The membrane was crosslinked twice with ultraviolet and pre-hybridized overnight at 40 °C with 10 ml of hybridization buffer (1 × SSC, 1% SDS, 200 μg ml −1 single-stranded DNA). A northern probe was prepared using the mir Vana miR Probe Construction Kit (Life Technologies). In the first step, a double-stranded DNA template for T7 transcription was generated according to the manufacturer’s instructions. The probe was denaturated at 95 °C for 1 min, placed on ice and hybridized against the membrane for 2 h at 40 °C in 10 ml of hybridization buffer. Subsequently, the membrane was washed two to three times for 30 min each with 50 ml of wash buffer (0.2% SSC, 0.2% SDS). The signal was registered with a radiographic film or exposed to a phosphoimaging screen and scanned on a FLA-5100 scanner (Fujifilm). Western blot analysis Total protein samples (100 μg per lane), isolated by sonication, were resolved by standard NuPAGE SDS–PAGE electrophoresis with MOPS running buffer (Life Technologies) and transferred onto nitrocellulose membrane. The membrane was blocked overnight at 4 °C with 1:10 western blocking reagent (Roche) in TBS buffer with 0.1% of Tween-20 (TBST). The following day, the membrane was incubated for 1 h at room temperature with primary antibody solution in 1:20 western blocking reagent diluted in TBST: rabbit polyclonal anti-Lin28a (A177) (1:1,000, Cell Signalling Technology), rabbit polyclonal anti Msi1 (N3C3) (1:1,000, GeneTex), rabbit monoclonal anti-hnRNP A1 (1:1,000, D21H11) (Cell Signalling Technology), Lin28b (1:1000, Cell Signalling Technology), Tuj1 (1:20,000, GeneTex), GFAP (1:1,000, SIGMA), DHX9 (1:1,000, Protein-Tech), mouse-monoclonal anti-β-tubulin (1:10,000, Sigma). After washing in TBST, the blots were incubated with the appropriate secondary antibodies conjugated to horseradish peroxidase and detected with SuperSignal West Pico detection reagent (Thermo Scientific). The membranes were stripped using ReBlot Plus Strong Antibody Stripping Solution (Chemicon) equilibrated in water, blocked in 1:10 western blocking solution in TBST and re-probed as described above. Full scans of the western blots presented in the manuscript are shown in the Supplementary Fig. 10 . In vitro processing assays Pri-miRNA and pre-miRNA substrates were prepared by standard in vitro transcription with T7 RNA polymerase in the presence of [α- 32 P]-UTP. Where indicated, pre-miRNA probes were 5′-end-labelled with [γ- 32 P]-ATP. The templates used to generate the transcripts were prepared by PCR amplification from cloned fragments of the human genome using corresponding primers ( Supplementary Table 2 ). Pri-miR-9-1/miR-16 TL and pri-let-7a-1/miR-16 TL templates were prepared based on mutagenesis of the wild-type pri-miR plasmids by replacing the terminal loops with the terminal loop from the miR-16 using corresponding primers ( Supplementary Table 2 ). Gel-purified probes (50 × 10 3 c.p.m. (counts per minute), ~20 pmol) were incubated in 30 μl reaction mixtures containing 50% (v/v) total P19 cell extracts (~10 μg μl −1 ), 0.5 mM ATP, 20 mM creatine phosphate and 3.2 mM MgCl 2 . Reactions were incubated at 37 °C for 30 min followed by phenol-chloroform extraction, precipitation and 8% (w/v) denaturing gel electrophoresis. In the case of pre-miRNA processing, 0.25 mM UTP was added to the reaction mixture. The signal was registered with a radiographic film or exposed to a phosphoimaging screen and scanned on a FLA-5100 scanner (Fujifilm). EMSA EMSA was performed with internally labelled pre-miR transcript and whole-cell extracts. Gel-purified probes (50 × 10 3 c.p.m., ~20 pmol) were incubated in 30 μl reaction mixtures containing 50% (v/v) total P19 cell extracts (~10 μg μl −1 ), 0.5 mM ATP, 20 mM creatine phosphate and 3.2 mM MgCl 2 . Reactions were incubated at 4 °C for 1 h followed by electrophoresis in 6% (w/v) non-denaturing gel. Where indicated, antibodies were added to reactions mixtures (1:100) to generate super shift. The signal was registered with a radiographic film or exposed to a phosphoimaging screen and scanned on a FLA-5100 scanner (Fujifilm). RNA pull down and mass spectrometry RNA pull down and mass spectrometry were performed as described previously [28] . In brief, total protein extracts from undifferentiated or differentiated P19 cells grown in ‘light’ [ 12 C]Arg/[ 12 Lys] and ‘heavy’ [ 13 C]Arg/[ 13 C]Lys isotopes, respectively, were incubated with synthesized RNAs, chemically coupled to agarose beads. All synthetic RNAs used are listed in Supplementary Table 3 . The incubation was followed by a series of washes with Roeder D buffer (100 mM KCl, 20% (v/v) glycerol, 0.2 mM EDTA, 100 mM Tris pH 8.0). After the final wash, the beads with associated proteins were re-suspended in structure buffer (10 mM Tris–HCl pH 7.2, 1 mM MgCl 2 , 40 mM NaCl) followed by treatment with RNAses. The samples were subsequently analysed by SDS–PAGE followed by mass spectrometry or western blot. RNAseq and small RNAseq Ten micrograms of total RNA was isolated from d0 and d4 P19 cells and analysed on the Illumina HiSeq2000 platform. Sample processing and analysis were preformed by BGI genomics. Data visualization was based on the bigwig files implemented into Ensembl Genome Browser. RNA interference and miR overexpression Pools of siRNAs were obtained from Dharmacon in the format of three independent siRNAs targeting different regions of the mRNA coding for the protein of interest. Genomic fragment containing miRs were cloned in pCG T7 plasmid and transiently expressed in P19 cells. Four micrograms of siRNAs was delivered in two transfection events separated by 48 h using nucleofection technology (AMAXA), according to the manufacturer instructions. Two micrograms of PCG T7 plasmids expressing miRs was delivered using similar methodology. For HeLa cells transfections were performed using Lipofectamine 2000 (Life Technologies), according to the manufacturer’s instructions. Stable cell line generation P19 cell lines with stable Lin28a-GFP or GFP only expression were gifts from Dr Eric Moss (The University of Medicine and Dentistry, NJ) [35] . Both lines were maintained in standard culture conditions. A P19 cell line expressing untagged Lin28a was developed using the Flp-in system (Life Technologies), according to the manufacturer’s instructions. In brief, the FRT site was randomly integrated in the genome and its integration was verified using Zeocin and lacZ selection markers. The Lin28a cDNA was integrated into the FRT site using Flp-mediated recombination and the event was confirmed using hygromycin selection as well as western blotting analysis. A P19 cell line with Tet-On 3G inducible expression of Lin28a was generated according to the manufacturer’s instructions (Clontech Lab Inc.). In brief, a pCMV-Tet3G plasmid coding for a Dox-responsive transactivator was integrated into undifferentiated P19 cells using a G418 selection marker. A pTRE3G-Bi-Luc plasmid expressing luciferase under a control transactivator-responsive promoter was used to select stable clones with high response to Dox (100 ng ml −1 ) treatment. Next, Lin28a was cloned to a pTRE3G-Bi plasmid and integrated into P19 cells with an active pCMV-Tet3G system using a linear hygromycin selection marker. Selected clones were expanded and differentiated using RA, as described above. On day 8 of differentiation, cells were induced with Dox (100 ng ml −1 ). The expression of Lin28a was checked at day 9 of differentiation. How to cite this article: Nowak, J. S. et al . Lin28a regulates neuronal differentiation and controls miR-9 production. Nat. Commun. 5:3687 doi: 10.1038/ncomms4687 (2014).